Synthesis of metalla-dual-azulenes with fluoride ion recognition properties 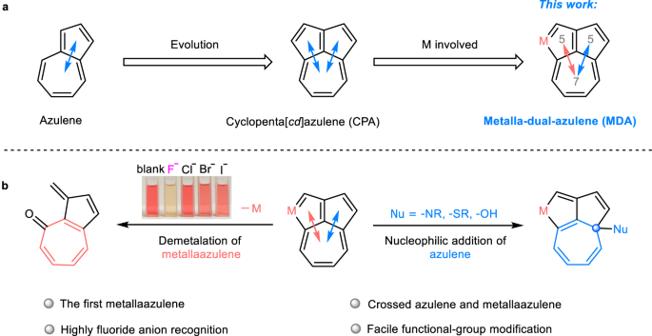Fig. 1: Overview of this work. aStructural skeletons of azulene, cyclopenta[cd]azulene (CPA) and metalla-dual-azulene (MDA).bThe reactivities of MDA, demetalation of MDA by treatment withnBu4NF along with the noticeable color change of the solution (left), and nucleophilic addition of MDA with various reagents (right). Azulene-based conjugated systems are of great interests due to their unusual structures and photophysical properties. Incorporation of a transition metal into azulene skeleton presents an intriguing opportunity to combine the d π - p π and p π - p π conjugated properties. No such metallaazulene skeleton however has been reported to date. Here, we describe our development of an efficient [5 + 2] annulation reaction to rapid construction of a unique metal-containing [5-5-7] scaffold, termed metalla-dual-azulene (MDA), which includes a metallaazulene and a metal-free organic azulene intertwined by sharing the tropylium motif. The two azulene motifs in MDA exhibit distinct reactivities. The azulene motif readily undergoes nucleophilic addition, leading to N-, O- and S-substituted cycloheptanetrienyl species. Demetalation of the metallaazulene moiety occurs when it reacts with n Bu 4 NF, which enables highly selective recognition of fluoride anion and a noticeable color change. The practical [5 + 2] annulation methodology, facile functional-group modification, high and selective fluoride detection make this new π-conjugated polycyclic system very suitable for potential applications in photoelectric and sensing materials. In the more than two centuries since the first aromatic compound, naphthalene was discovered, there has been a continuous interest in the synthesis and research of the properties of various fused-ring skeletons. Azulene is a non-benzenoid hydrocarbon isomer of naphthalene that has attracted significant attention from chemists because of its unique properties and reactivities which arise from the fusion of an electron-rich 5-membered ring and an electron-deficient 7-membered ring, producing a compound with a dipole moment of 1.08 D [1] , [2] . This structure has been used extensively for the construction of azulene-based π-functional materials, polycyclic aromatic hydrocarbons, and heteroaromatics [3] , [4] , [5] . Cyclopenta[ cd ]azulene (CPA), a [5-5-7] fused-tricyclic framework that consists of two azulene moieties fused to the same 7-membered ring is of particular interest (Fig. 1a ). It was first synthesized by Hafner et al. in 1959 [6] and its structure was subsequently confirmed in 1970 [7] . Only a few synthetic methods and reactivity studies concerning CPA have since been reported [8] , [9] , [10] , [11] , [12] , [13] , but because the tricyclic [5-5-7] skeleton and its derivatives have been found in fullerenes [14] , [15] , nanographenes [16] , [17] , natural products and drug-like molecules [18] , [19] , designing and exploring the reactivity of the [5-5-7] skeleton is of great significance. Fig. 1: Overview of this work. a Structural skeletons of azulene, cyclopenta[ cd ]azulene (CPA) and metalla-dual-azulene (MDA). b The reactivities of MDA, demetalation of MDA by treatment with n Bu 4 NF along with the noticeable color change of the solution (left), and nucleophilic addition of MDA with various reagents (right). Full size image Metal-containing polycyclic π-conjugated systems continue to attract considerable attention [20] , [21] , [22] , [23] . The incorporation of transition metal with d -orbitals into the organic polycyclic framework results in d π – p π -conjugated patterns, providing both organic and organometallic characteristics and leading to special physicochemical properties and possible applications [24] . In recent decades, significant progress has been made in the development of polycyclic metallacycles with 5-membered or 6-membered ring motifs [25] , [26] , [27] , [28] , including metalla-naphthalene [29] , [30] , metallaanthracene [31] , [32] , metallapentalenes [33] , [34] , and other motifs [35] , [36] , [37] . However, hydrocarbon seven-membered ring, especially the azulene motif, has not been observed in these polycyclic metallacyclic systems, notwithstanding a few reports of metallacyclo-heptatrienes [38] , [39] , [40] . Further research could potentially lead to the discovery of new compounds with unique properties and reactivities. Herein, we present a convenient [5 + 2] annulation strategy which can be used to construct an uncommon metal-containing [5-5-7] skeleton termed a metalla-dual-azulene (MDA). This structure can be viewed as a cross between a metallaazulene and an organic azulene, with both sharing a seven-membered ring (Fig. 1a ). The replacement of a carbon by a transition metal in the [5-5-7] skeleton can have a significant impact on the dipole moment of the molecule, and shows that the two azulene fragments exhibit completely different reactivities. The organic azulene motif allows for facile installation of various substituents in the 7-membered ring through nucleophilic addition, providing a wide range of functional group diversity and fine-tuning of the compounds’ electronic properties (Fig. 1b , right). Demetalation of the metallaazulene moiety can be achieved by treatment with n Bu 4 NF, leading to a distinct and visible color change. This recognition of a fluoride ion is not impeded in any of the twelve different anions, and the limit of detection (LOD) of fluoride has been determined to be 9.73 × 10 -7 M (18.44 ppb), thereby providing a sensitive method for detection of fluoride ions in solution (Fig. 1b , left). Synthesis of precursor (1) and preparation of metalla-dual-azulene compounds (2a–2h) by [5 + 2] annulation of 1 with alkynes Treatment of the diyne ( L ) with [Ir(CH 3 CN)(CO)(PPh 3 ) 2 ]BF 4 in CH 2 Cl 2 under N 2 at r.t. for 6 h resulted in the formation of compound 1 with an isolated yield of 81% (Fig. 2a ). Single-crystal X-ray analysis indicated that 1 contains a tricyclic skeleton of an iridacyclopentadiene fused two rings (Fig. 2c ). A possible mechanism for the formation of 1 , involving the [2 + 2 + 1] cycloaddition of L with a simple metal complex is proposed (Supplementary Information—p. 9 ). Fig. 2: Synthesis and characterization of precursor 1 and compounds 2a–2h. a and b Synthesis of compound 1 and preparation of 2a – 2h by reactions of 1 with different alkynes. c X-ray structures for the cations of compounds 1, 2a – 2d (thermal ellipsoids drawn with 50% probability, the phenyl groups in PPh 3 and isopropyl groups in −CH = N + ( i Pr) 2 were omitted for clarity) and the selected bond lengths (Å) for 2a – 2d . Selected bond distances (Å) for 1 : Ir1–C1 2.183(4), Ir1–C7 2.139(4), C1–C2 1.362(6), C2–C6 1.447(5), C6–C7 1.362(6), C2–C3 1.468(6), C3–C4 1.398(6), C4–C5 1.519(6), C5–C6 1.530(6). Full size image Compound 1 contains a bent phenyl allyl alcohol fragment, which serves as a five-carbon synthon with potential reactivity toward unsaturated substrates. Accordingly, treatment of 1 with phenylacetylene and AgBF 4 in the presence of HBF 4 ·Et 2 O at r.t. in CH 2 Cl 2 for 15 min led to the formation of compound 2a with an isolated yield of 87% (Fig. 2a ). The reaction involves a formal [5 + 2] cycloaddition of the phenyl allyl alcohol in 1 with phenylacetylene, constructing a seven-membered ring, and leading to the formation of a π-conjugated fused pentacyclic iridium compound. To investigate the generality of this reaction, various alkynes with different groups were investigated (Fig. 2b ). Phenylacetylene with an electron-donating (–OMe) substituent or an electron-deficient group (–CF 3 ) at the para -position proved to be good substrates, giving the corresponding products in good yields (90% for 2b , 85% for 2c ). 4-Ethynylbiphenyl, naphthylene-2-acetylene, and 3-ethynylthiophene were also tolerated well and afforded the targeted product ( 2d – 2f ) in good yields. The internal alkynes, 1-phenyl-1-propyne, and 1-phenyl-1-pentyne also reacted smoothly, affording the desired products in excellent yield (82% for 2g , 84% for 2h ). Both aryl-substituted terminal and internal alkynes are well compatible in the reactions, however, when substituting the alkynes with alkyl groups (e.g. 1-heptyne, ethoxyethyne, and 3-butyn-2-one), there are no products observed (Supplementary Information, pp. 37 – 38 ). Single-crystal X-ray diffraction analysis revealed that compounds 2a – 2d contain an extended π-conjugate pentacyclic system, comprised of a [5-5-7] tricyclic iridacycle fused with one phenyl ring and attached to a second phenyl ring (Fig. 2c and Supplementary Information, pp. 45 – 48 ). The central [5-5-7] skeleton can be regarded as a metallaazulene combined with an organic azulene by sharing the seven-membered ring, resulting in a unique metalla-dual-azulene compound such as 2a – 2d . The Ir–C bond lengths in 2a (Ir1–C1: 2.115(11) Å, Ir1–C10: 2.182(9) Å) are almost identical, while the C–C bond lengths within the two fused five-membered rings (1.351(14)–1.478(13) Å) and the newly formed seven-membered ring (1.392(14)–1.442(14) Å) are intermediate between typical C–C single and C=C double bond lengths [23] , [35] , [41] , indicating a delocalized [5-5-7] structure. The seven-membered ring is almost planar, as reflected by the mean deviation of 0.086 Å from the least-squares plane. The C–C bond distances and the planarity suggest it is an aromatic tropylium motif [42] , indicating a significant contribution from the resonance form 2 ’. The structures of compounds 2a – 2h were also confirmed by nuclear magnetic resonance spectroscopy (NMR) and high-resolution mass spectrometry (HRMS) (Supplementary Information, pp. 9 – 15 ). The signal from the proton at C6 in 2a was observed at δ = 6.69 ppm in the aromatic proton region, showing a distinct shift to the lower field when compared to traditional alkenes. In the 13 C{ 1 H} NMR spectrum of 2a , the signal (227.3 ppm) from C10 was observed at a significantly lower field than that of C1 (176.6 ppm). This is probably because C10 is situated in a positive tropylium environment, which further suggests the resonance contribution of 2 ’. The 31 P{ 1 H} NMR spectrum shows only a singlet at −2.6 ppm, attributed to IrPPh 3 . Experimental and theoretical investigations of the mechanism Control experiments were conducted to elucidate the mechanism of the reaction, including the identification of key intermediates and the detection of hydrogen. Stepwise addition of HBF 4 ·Et 2 O and AgBF 4 was performed to examine their respective roles in the reaction. First, treatment of 1 and phenylacetylene with HBF 4 ·Et 2 O at r.t. in CH 2 Cl 2 resulted in a 93% yield of a new compound ( 3a ) (Fig. 3a ). The X-ray crystal structure of 3a shows that it has a pentacyclic skeleton similar to that of 2a , except that the seven-membered ring is a cycloheptatrienyl motif. This is confirmed by the typical C–C single bond lengths of C11–C5 (1.509(6) Å) and C5–C6 (1.501(7) Å) (Fig. 3b ). The signal attributed to the hydrogen at C5 was observed at δ = 3.28 ppm in the 1 H NMR spectrum. Subsequently, treatment of the isolated 3a with AgBF 4 in CH 2 Cl 2 led to the corresponding compound ( 2a ) in 89% yield. Hydrogen produced in the in situ reaction was detected by gas chromatography (GC) (Fig. 3b right), and the formation of silver mirrors was observed after the reaction (Supplementary Information, p. 16 ). These results suggest the reaction initially proceeds through [5 + 2] cycloaddition promoted by HBF 4 ·Et 2 O to form a cycloheptatrienyl intermediate, which then undergoes oxidative dehydrogenation enabled by AgBF 4 . The latter process can also proceed in the presence of other oxidants, such as MnO 2 or AgOTf. Fig. 3: Control experiments and proposed mechanism. a Isolation of intermediate 3a and its further conversion to 2a by stepwise addition of HBF 4 ·Et 2 O and AgBF 4 in the reaction. b Structure of the cation of 3a (thermal ellipsoids drawn with 50% probability, the phenyl groups in PPh 3 and isopropyl groups in −CH = N + ( i Pr) 2 omitted for clarity) (left), selected bond lengths (Å) for 3a (middle), detection of H 2 by GC (gas chromatography) in the conversation of intermediate 3a to 2a (right). c Proposed mechanism for the formation of 2a . Full size image Based on these experimental results, a plausible mechanism was proposed for the formation of 2a (Fig. 3c ). The process begins with the dissociation of the hydroxyl group in 1 by HBF 4 ·Et 2 O, giving Int1 . Next, the electrophilic addition of Int1 to phenylacetylene affords vinyl cation Int2 , which is a common intermediate observed in alkynes participating reactions [43] , [44] , [45] . Subsequently, intramolecular electrophilic attack within Int2 generates a [5 + 2] annulated cation species Int3 . The loss of a proton from the cation completes the Friedel–Crafts cyclization, resulting in the formation of stable 3a . Finally, oxidative hydride abstraction of 3a by AgBF 4 affords the target product ( 2a ). Further evidence for the proposed mechanism involving electrophilic addition via Int2 has been provided and directly calculating the [5 + 2] cyclization pathway has been ruled out (Supplementary Information, pp. 37 – 38 ). Development of efficient and straightforward methods for constructing seven-membered rings has practical significance. Previously reported methods for construction of 7-membered rings via [5 + 2] cycloaddition have utilized vinylcyclopropanes [46] , [47] , [48] , 3-acyloxy-1,4-enynes [49] , [50] and metal η 5 -pentadienyl compounds [51] as the five-carbon synthons. However, methods to synthesize tropylium ions are relatively limited and often require multiple reactions [52] , [53] , [54] . In this case, [5 + 2] cycloaddition via a Friedel–Crafts cyclization and aromatization provides a new and efficient route with which to build the tropylium motif. The use of an iridacyclopentadiene derivative ( 1 ) as the five-carbon synthon enables access to a new metal-incorporated [5-7] bicyclic skeleton, which is an unprecedented metallaazulene motif. DFT calculations were conducted to gain a deeper understanding of the mechanism. The computed Gibbs free energy profile of the essential reaction steps is shown in Fig. 4 . In the HBF 4 ·Et 2 O promoted reaction, the conversion of reactant 1 to Int3 is energetically favored and achieved smoothly with no high barriers lowering the potential energies. Two possible pathways can lead from Int3 to product 2a . The direct formation of 2a through TS3 ’ has a high barrier of 19.3 kcal mol −1 (Fig. 4 , gray line). In contrast, the formation of intermediate 3a through TS3 is kinetically favored, with a negligible barrier of 0.1 kcal mol −1 , and results in the formation of stable compound ( 3a ) with an exothermicity of 18.2 kcal mol −1 (Fig. 4 , black line). The oxidative dehydrogenation of 3a by AgBF 4 affords the 7-membered ring in the final product 2a . The aromaticity of this 7-membered motif has been evaluated by calculated results of the nucleus-independent chemical shift (NICS) values and the anisotropy of the current-induced density (ACID) (Supplementary Information, p. 35 ). Fig. 4: DFT calculations for mechanistic investigation. Gibbs free energy profile for the formation of compounds 3a and 2a . Energies are given in kcal mol −1 . The Gibbs free energy of reactant 1 with HBF 4 ·Et 2 O was designated as 0 kcal mol −1 . The B3LYP-D3BJ/Def2-TZVP method with the SMD solvation method in CH 2 Cl 2 was used. Full size image Nucleophilic addition of metalla-dual-azulene with versatile –N, –S, and –O reagents The presence of a cationic tropylium moiety in metalla-dual-azulene makes it susceptible to nucleophilic reactions. Indeed, treatment of 2a with NaOH in CH 2 Cl 2 for 15 min resulted in the formation of a product ( 4a ) in high yield (96%) (Fig. 5a ). The X-ray crystal structure of 4a revealed a pentacyclic skeleton with a hydroxyl group attached at C5. The bond lengths of C5–C11 (1.513(6) Å) and C5–C6 (1.494(6) Å) indicate the typical C–C single bonds (Fig. 5b and Supplementary Information, p. 49 ). The 7-membered ring is extremely torsional, as reflected by the large mean deviation of the least-squares plane (0.303 Å), in contrast to the high planarity of the precursor 2a (0.086 Å). Nucleophilic addition to the tropylium species resulted in the formation of a cycloheptatrienyl motif. Notably, compound 4a can be efficiently transferred back to 2a by treating with HBF 4 ·Et 2 O (Supplementary Information, p. 27 ). The result indicates that the reversible conversion between compounds 2a and 4a can be achieved by regulating the acidity and basicity of the system. Other nucleophiles, including aniline, sodium thiomethoxide, and sodium thiophenoxide were also reacted with 2a , and the desired products ( 5a, 6a , and 6b ) were obtained in 95%, 90%, and 81% yields, respectively. A condensed dual descriptor (CDD) study showed that both C5 and C7 sites are electron-deficient (Supplementary Information, p. 35 ). We performed further calculations to evaluate the main contributions of resonance structures ( 2a-I – 2a-IV ) with positive charge distribution on the seven-membered ring (7MR) using the natural resonance theory analysis method (NRT). The results revealed that resonance structure 2a-I with the positive charge on C5 had the highest contribution, accounting for a maximum proportion of 22.53% compared to other structures ( 2a-I – 2a-IV ), which explains the nucleophilic addition occurred exclusively at the C5 site (Supplementary Information, p. 36 ). Fig. 5: The reactivities study of 2a and the direct synthesis of compounds 4a–4j. a Nucleophilic addition of 2a with versatile nucleophiles (NaOH, PhNH 2 , and NaSR”). b X-ray structures for 4a, 6a , and 6b (drawn with 50% probability level) and the selected bond lengths (Å). c Direct synthesis of –OH substituted products 4a – 4j by reaction of 1 with various alkynes. Full size image A direct and convenient route to form 4a was developed, starting from 1 which was treated with phenylacetylene and HBF 4 ·Et 2 O with AgBF 4 at r.t. in CH 2 Cl 2 for 15 min. The mixture was filtered and concentrated, and then subjected to chromatography on a basic alumina column, giving compound 4a with an isolated yield of 85%. An 18 O labeling experiment showed that the hydroxyl group (– 18 OH) attached to C5 of compound 4 originated from the H 2 O in the system, which was confirmed by HRMS (Supplementary Information, pp. 25 – 26 ). Different alkynes with various functional groups were investigated (Fig. 5c ). Phenylacetylenes bearing electron-donating substituents (–Me, – t Bu, or –OMe) at para -positions were shown to be excellent substrates, giving the corresponding products ( 4b, 4c , and 4d ) in yields of 89%, 90%, and 91%, respectively. Electron-withdrawing groups (–CF 3 ) or halogen (–F) and (–Ph) substituents at para -positions or meta -positions also demonstrated good applicability as substrates with yields of 89%, 85%, and 87% for 4e, 4f , and 4g , respectively. The polycyclic 1-naphthylethyne and heterocyclic 2-ethynylthiophene reacted smoothly and afforded the desired products 4h and 4i in 89% and 61% yields, respectively. The internal alkyne (1-phenyl-1-propyne) was also compatible and gave the corresponding product ( 4j ) with an 86% yield. The structures of all the compounds ( 4a – 4j ) were confirmed by NMR spectroscopy, HRMS, and the structures of 4a, 4d, 4f , and 4j were further confirmed by X-ray diffraction (Supplementary Information, pp. 49 – 52 ). UV–Vis absorption spectra of products and fluoride anion recognition properties of 2a The UV–Vis absorption spectra showed that the pentacyclic compounds all exhibit strong absorption bands. As depicted in Fig. 6a , the characteristic energy absorption band of 2a in the low-energy absorption regions (537 nm) is red-shifted by ~39 nm compared to the precursor 1 (498 nm) due to the extended π-conjugated framework in 2a . The molar absorption coefficient of 2a at 537 nm is 1.4 × 10 4 M −1 cm −1 . The characteristic energy absorption could be fine-tuned by modifying the substituents on the seven-membered ring. Specifically, the electron-donating group (–OMe) in R 1 of 2b resulted in a significantly red-shifted absorption at 565 nm when compared with compound 2c , which contains an electron-withdrawing group (–CF 3 ) (528 nm). The absorption spectra of dearomatized counterparts ( 4a, 5a, 6a , and 6b ) exhibited similar absorption properties (Fig. 6a right), but the molar absorption coefficient value ( ε ) of characteristic energy absorption varied from 1.4 to 1.9 × 10 4 M −1 cm −1 . Fig. 6: Optical properties and fluoride anion recognition. a UV–Vis absorption spectra of compounds 1, 2a – 2h, 4a, 5a, 6a , and 6b measured in CH 2 Cl 2 at r.t. (1.0 × 10 -5 M). b Selected highest occupied molecular orbitals (HOMO) and lowest unoccupied molecular orbitals (LUMO) related to the excitation of compound 2a and 4a (isovalue = 0.02) are given. The eigenvalues of the MOs (molecular orbitals) are given in parentheses. c Excited wavelength ( λ ) oscillator strengths ( f ) and related wavefunctions. d Color changes of 2a (0.07 mM) by the addition of 5.0 equiv. of various anions (0.35 mM) including F − , Cl − , Br − , I − , ClO 4 − , NO 3 − , NO 2 − , PF 6 − , HSO 4 − , SO 4 2− , TfO − , HCO 3 − and CO 3 2− of n Bu 4 NX salts in CH 2 Cl 2 for 5 min, respectively. e Mixing the solutions with each of the above 12 anions (left) and without the addition of F − (right). f UV–Vis absorption spectra of 2a (0.07 mM) after the addition of 5.0 equiv. of different anions in CH 2 Cl 2 . g Linear relationship for absorbance at 515 nm for 2a versus the concentration of n Bu 4 NF (7.0–35 μM). h The in situ UV–Vis absorption of 2a (0.07 mM) and n Bu 4 NF (5.0 equiv.) in CH 2 Cl 2 was monitored within 2.5 h. i Isolation of product 7a by reaction of 2a with n Bu 4 NF. X-ray structures for 7a (drawn with 50% probability level). j UV–Vis absorption spectra of 2a and 7a in CH 2 Cl 2 and the corresponding photographs of solutions (inset). Full size image To further analyze the absorption spectra, we implemented time-dependent DFT calculations at the B3LYP-D3BJ/Def2-TZVP level for compounds 2a and 4a (Fig. 6b, c ). The calculated excited wavelength λ max = 515 nm of 2a was found to be 95.8% attributable to HOMO → LUMO transitions, with a corresponding oscillator strength ( f ) of f = 0.2561. Meanwhile, the calculated excited wavelength λ max = 509 nm of 4a was found to be 97.4% attributable to HOMO → LUMO transitions, with a corresponding oscillator strength of f = 0.2414. Notably, the nucleophilic addition to the tropylium motif in 2a led to the formation of a cycloheptatrienyl motif with a C( sp 3 ) site in 4a . However, despite this change, the electron delocalization of 4a remains similar to that of 2a over the polycyclic skeletons. Additionally, their HOMO–LUMO gap is nearly identical (Δ Ε = 2.88 eV for 2a , Δ Ε = 2.89 eV for 4a ). This explains the similarity of the absorption maxima of 2a and 4a in the low-energy absorption regions. The theoretical spectra are thus consistent with the trends observed in the experimental spectra. The electrochemical properties of these pentacyclic compounds have also been investigated. The complexes exhibit redox processes, however, are found to be irreversible (Supplementary Information, p. 40 ). Compounds 2a – 2h in the solid state are all stable below 130 °C in air for at least 4 h (Supplementary Information, p. 41 ). They have a cationic tropylium motif and strong absorptions in the visible range, which led us to explore their potential as colorimetric chemosensors through interactions with anions. Upon adding 5.0 equiv. of tetra- n -butylammonium salts ( n Bu 4 NX), including X = Cl − , Br − , I − , ClO 4 − , NO 3 − , NO 2 − , PF 6 − , HSO 4 − , SO 4 2− , TfO − , HCO 3 − , and CO 3 2− to a solution of 2a , weak or negligible color changes were observed for these anions. However, when mixed with fluoride anion (F − ), a rapid and obvious change to essentially colorless occurred within 5 min (Fig. 6d ). The UV–Vis absorption spectra showed a significant decrease in the absorption bands around 515 nm in the presence of fluoride anion (Fig. 6f ). The solutions displayed no noticeable color change when 2a was added to a mixture of 12 anions without F − (Fig. 6e , right), but the color faded immediately upon addition of F − to the anionic mixture (Fig. 6e , left). These results indicate that 2a has promising selective recognition of F − in an organic solvent, and is not affected by other anions. Based on the results from the absorbance titration, it was concluded that the detection limitation of 2a for fluoride anion was sensitive. A linear curve was fitted showing the decreased absorbance versus the concentration of F − ranging from 7.0 to 35 μM under the same sensing conditions (Fig. 6g ). The limits of detection (LOD) were calculated as 3 σ / k , where k is the slope of the linear fitting and σ is the standard deviation of blank measurements. It was found that 2a had a detection limit of 9.73 × 10 −7 M (18.44 ppb) for F − , implying a highly sensitive detection ability (Fig. 6g and Supplementary Information, pp. 32 – 33 ). The in-situ UV–Vis spectroscopy showed that the characteristic absorption peak at ~515 nm decreased gradually over 2.5 h when 5.0 equiv. F − was added (Fig. 6h ). These results suggest that 2a can detect F − through color changes that are easily observed with the naked eye or by colorimetric measurement. As fluoride ions are commonly present in aqueous solutions, we conducted further investigations to evaluate the effect of water on the recognition of fluoride ions. By adding different amounts of water (0.01–2.0 mL) into the reaction systems containing 2a and n Bu 4 NF, the color of the solution changed rapidly from red to light yellow, which was similar to the observation in the blank reaction where no water was added. The UV–Vis absorption spectra of the resulting solutions also exhibit no significant changes compared to the blank sample (Supplementary Information, p. 33 ). The findings indicated that the fluoride ion recognition capacity off. To investigate the nature of the specificity of 2a towards F − , we conducted experiments to isolate the product of the reaction of 2a with n Bu 4 NF and succeeded in obtaining a product ( 7a ). The X-ray crystal structure of 7a revealed that it is an organic tetracyclic framework without the iridium fragment (Fig. 6i ). An 18 O labeling experiment showed that the oxygen atom of the carbonyl group (C=O) attached to C10 in compound 7a originates from the H 2 O present in the system (Supplementary Information, p. 31 ). In the presence of n Bu 4 NF, demetalation of 2a may be triggered by the interaction of the fluoride anion with the metal center, subsequently inducing the demetalation process (Supplementary Information, p. 32 ). Fluoride ion is considered less nucleophilic in comparison to –O, –N, and –S nucleophilic reagents (Fig. 5a ), therefore, fluoride ion does not proceed through direct nucleophilic addition in this case. Notably, retention of 2a for other n Bu 4 NX salts (X = Cl, Br, I) as evidenced by there being essentially no change in the UV–Vis spectra. Consistently, previous research has shown that the tropylium moiety is capable of detecting fluoride ions out of its halide family [55] . The development of fluoride probes is of considerable significance in health and environmental issues [56] , [57] , and previously reported F − sensors have been designed based on the interactions between fluoride anions and Lewis acids, fluoride–hydrogen bonding [58] , fluoride–silicon bond interaction, and other types of materials [59] , [60] . In the present case, a new reaction-based colorimetric fluoride sensor involving demetalation has been developed, leading to color responses that allow for detection by the naked eye (Fig. 6j ). The metal interacting with a conjugated system enables a significant enhancement of the absorption and color change, which is a prerequisite for detection. We have developed an efficient [5 + 2] annulation reaction to rapidly build a unique metal-containing [5-5-7] scaffold, known as metalla-dual-azulene. This is composed of a metallaazulene and an organic azulene that share the tropylium motif. The reaction involves a Friedel–Crafts cyclization and oxidative dehydrogenation under mild conditions. The resulting fused-polycyclic metallacycles exhibit strong absorption bands in the UV–Vis spectra, with characteristic energy absorption bands that can be finely tuned by modifying the substituents at C5, C6, and C7 on the seven-membered ring. In a mixture of 13 available anions, the metalla-dual-azulene ( 2a ) demonstrates highly selective recognition of the fluoride anion with noticeable color changes that allow for detection by the naked eye. The findings of this study offer a valuable strategy for the construction of seven-membered rings and create new opportunities for enlarging the π-conjugated polycyclic systems with fascinating properties. General information Details of the synthesis and characterization of the multiyne ( L ) and metallapolycyclic compounds ( 1, 2a–2h, 3a, 4, 5a, 6a, 6b , and 7a ) can be found in the supplementary information, pp. 5 – 31 . For X-ray data of all the described compounds ( L, 1, 2a–2d, 3a, 3x, 4a, 4d, 4f, 4j, 6a, 6b, and 7a ) see supplementary information, pages 42 - 67 . For HRMS, 1 H, 31 P{ 1 H} NMR, and 13 C{ 1 H} NMR spectra of compounds in this article, see Supplementary Information, pp. 69 – 117 and Supplementary Figs. 37 – 134 . For the thermal decomposition data of compounds 2a-2h, 3a, 4a, 5a, 6a , and 6b , see Supplementary Information, p. 41 . General procedure for preparation of compound 2 Alkyne (0.24 mmol) and HBF 4 ·Et 2 O (0.10 mmol) were added to a mixture of 1 (235.4 mg, 0.20 mmol) and AgBF 4 (116.4 mg, 0.60 mmol) in CH 2 Cl 2 (2.0 mL), which was stirred at r.t. under nitrogen for 15 min to give a brown solution. The solution was filtered through Celite, and the filtrate was concentrated under a vacuum. The resulting residue was purified by column chromatography (silica gel (200–300 mesh), eluent: dichloromethane/acetone = 2:1) to afford compounds 2 . General preparation procedure of compounds 4a, 5a, 6a, 6b A mixture of 2a (269.4 mg, 0.20 mmol) and 1.2 equiv. nucleophilic reagents (NaOH, PhNH 2 , NaSCH 3 , NaSPh, respectively) in CH 2 Cl 2 (2.0 mL) were stirred at r.t. under nitrogen for 2–6 h to give a pink solution. Then the solution was filtered by Celite, and the filtrate was concentrated under a vacuum. The resulting residue was purified by reverse precipitation performed with hexane or column chromatography (alumina (200–300 mesh) to afford the target product. 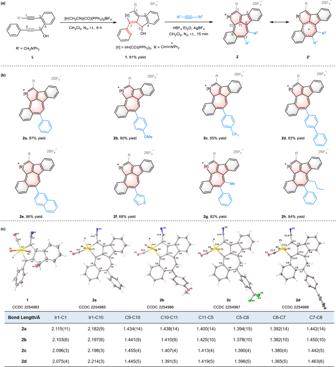Fig. 2: Synthesis and characterization of precursor 1 and compounds 2a–2h. aandbSynthesis of compound1and preparation of2a–2hby reactions of1with different alkynes.cX-ray structures for the cations of compounds1,2a–2d(thermal ellipsoids drawn with 50% probability, the phenyl groups in PPh3and isopropyl groups in −CH = N+(iPr)2were omitted for clarity) and the selected bond lengths (Å) for2a–2d. Selected bond distances (Å) for1: Ir1–C1 2.183(4), Ir1–C7 2.139(4), C1–C2 1.362(6), C2–C6 1.447(5), C6–C7 1.362(6), C2–C3 1.468(6), C3–C4 1.398(6), C4–C5 1.519(6), C5–C6 1.530(6). 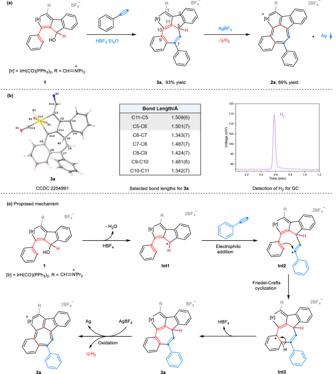Fig. 3: Control experiments and proposed mechanism. aIsolation of intermediate3aand its further conversion to2aby stepwise addition of HBF4·Et2O and AgBF4in the reaction.bStructure of the cation of3a(thermal ellipsoids drawn with 50% probability, the phenyl groups in PPh3and isopropyl groups in −CH = N+(iPr)2omitted for clarity) (left), selected bond lengths (Å) for3a(middle), detection of H2by GC (gas chromatography) in the conversation of intermediate3ato2a(right).cProposed mechanism for the formation of2a. 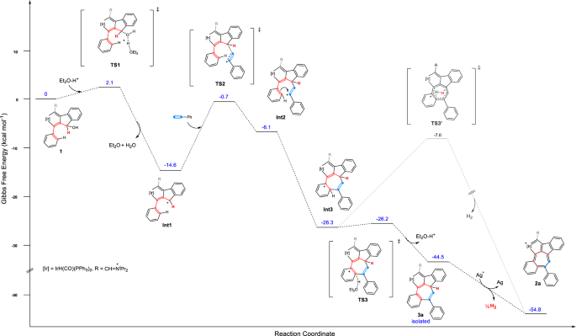Fig. 4: DFT calculations for mechanistic investigation. Gibbs free energy profile for the formation of compounds3aand2a. Energies are given in kcal mol−1. The Gibbs free energy of reactant1with HBF4·Et2O was designated as 0 kcal mol−1. The B3LYP-D3BJ/Def2-TZVP method with the SMD solvation method in CH2Cl2was used. 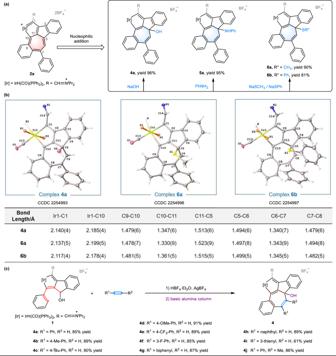Fig. 5: The reactivities study of 2a and the direct synthesis of compounds 4a–4j. aNucleophilic addition of2awith versatile nucleophiles (NaOH, PhNH2, and NaSR”).bX-ray structures for4a,6a, and6b(drawn with 50% probability level) and the selected bond lengths (Å).cDirect synthesis of –OH substituted products4a–4jby reaction of1with various alkynes. 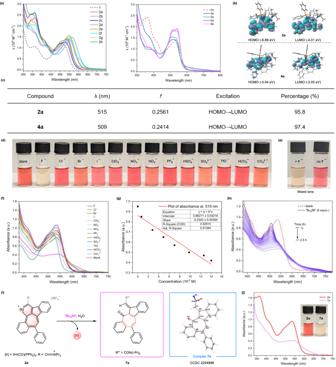Fig. 6: Optical properties and fluoride anion recognition. aUV–Vis absorption spectra of compounds1,2a–2h,4a,5a,6a, and6bmeasured in CH2Cl2at r.t. (1.0 × 10-5M).bSelected highest occupied molecular orbitals (HOMO) and lowest unoccupied molecular orbitals (LUMO) related to the excitation of compound2aand4a(isovalue = 0.02) are given. The eigenvalues of the MOs (molecular orbitals) are given in parentheses.cExcited wavelength (λ) oscillator strengths (f) and related wavefunctions.dColor changes of2a(0.07 mM) by the addition of 5.0 equiv. of various anions (0.35 mM) including F−, Cl−, Br−, I−, ClO4−, NO3−, NO2−, PF6−, HSO4−, SO42−, TfO−, HCO3−and CO32−ofnBu4NX salts in CH2Cl2for 5 min, respectively.eMixing the solutions with each of the above 12 anions (left) and without the addition of F−(right).fUV–Vis absorption spectra of2a(0.07 mM) after the addition of 5.0 equiv. of different anions in CH2Cl2.gLinear relationship for absorbance at 515 nm for2aversus the concentration ofnBu4NF (7.0–35 μM).hThe in situ UV–Vis absorption of2a(0.07 mM) andnBu4NF (5.0 equiv.) in CH2Cl2was monitored within 2.5 h.iIsolation of product7aby reaction of2awithnBu4NF. X-ray structures for7a(drawn with 50% probability level).jUV–Vis absorption spectra of2aand7ain CH2Cl2and the corresponding photographs of solutions (inset). Yield: 96% for 4a , 95% for 5a , 90% for 6a , 81% for 6b , respectively).